Muscle stem cells contribute to myofibres in sedentary adult mice Skeletal muscle is essential for mobility, stability and whole body metabolism, and muscle loss, for instance, during sarcopenia, has profound consequences. Satellite cells (muscle stem cells) have been hypothesized, but not yet demonstrated, to contribute to muscle homeostasis and a decline in their contribution to myofibre homeostasis to play a part in sarcopenia. To test their role in muscle maintenance, we genetically labelled and ablated satellite cells in adult sedentary mice. We demonstrate via genetic lineage experiments that, even in the absence of injury, satellite cells contribute to myofibres in all adult muscles, although the extent and timing differs. However, genetic ablation experiments showed that satellite cells are not globally required to maintain myofibre cross-sectional area of uninjured adult muscle. Skeletal muscle is critical for locomotion, structural support and regulation of whole body metabolism. Consequently, homeostatic maintenance of muscle mass is essential for muscle function, and pathological loss of muscle has profound negative consequences [1] . During aging, even in otherwise healthy individuals, muscle mass and function are progressively lost, in a process termed sarcopenia [1] , [2] . Sarcopenia strongly affects quality of life by impairing locomotion, increasing the likelihood for injury and increasing the risk of insulin resistance and type 2 diabetes [1] . Thus, an understanding of the requirements for maintaining muscle homeostasis is a critical human health need. Muscle is composed of multinucleate myofibres, and all myonuclei are terminally post-mitotic. Maintenance of muscle mass requires conservation of both the number and size of myofibres, and the number of myonuclei in a myofibre is an important regulator of myofibre size [3] . During sarcopenia, loss of muscle mass is due to both a loss of myofibres and a decrease in myofibres’ cross-sectional area (CSA), with fast contracting myofibres and hind limb muscles (in humans, mice and rats) being particularly vulnerable [1] , [4] . The mechanisms regulating muscle homeostasis and sarcopenia are complex and involve regulation of protein turnover by motor neurons, hormones, immune signals, nutrition and physical activity [1] . Adult muscle contains a population of resident stem cells, called satellite cells, and an important unresolved question is whether satellite cells play a role in muscle homeostasis and sarcopenia [4] , [5] , [6] , [7] . Genetic labelling and ablation studies have definitively established that satellite cells are the endogenous stem cells necessary and sufficient for muscle regeneration [8] , [9] , [10] and that they contribute to muscle hypertrophy as well [11] . In the absence of injury, satellite cells are thought to be quiescent and both myonuclear and myofibre number invariant [4] , but a limited number of studies indicate that new myonuclei are added to uninjured myofibres [12] , [13] , [14] . Because myonuclei are post-mitotic, this suggests that satellite cells contribute myonuclei during homeostasis. During aging, multiple studies show that myonuclei are lost [3] , [15] , [16] , [17] , leading to myofibre atrophy [3] , and suggest that in sarcopenia satellite cell replenishment of myonuclei may be inadequate. However, neither the hypothesis that satellite cells contribute to muscle homeostasis nor the hypothesis that a decline in satellite cell-mediated replenishment of myonuclei contributes to sarcopenia has been explicitly tested. In this study, we use mouse genetics to specifically label or ablate satellite cells to test their role in muscle homeostasis. We demonstrate via genetic lineage experiments that during adulthood satellite cells contribute to uninjured myofibres in all muscles, including hind limb, diaphragm and extraocular (EOMs) muscles. However, genetic ablation experiments showed that satellite cells are not globally required to maintain myofibre CSA of uninjured adult muscle. Satellite cell number differs between muscles and with age The number of satellite cells resident in a particular muscle is potentially an important determinant of a muscle’s ability to maintain homeostasis. Multiple studies report that satellite cells differ between anatomical muscles [18] , [19] , [20] , [21] , [22] , are enriched in muscles with slow MyHCI myofibres [17] , [19] , [20] , [22] , and vary with age [23] . Cross-comparison of these studies has been hampered by the use of different species at diverse ages, and the use of different satellite cell markers and methodologies for quantification. To date, no single study has compared the number of satellite cells in multiple muscles concurrently and over time. To explicitly compare satellite cell numbers in different muscles, we examined five hind limb muscles, the diaphragm and EOMs of adult male mice. We focused on hind limb muscles because these are highly susceptible to sarcopenia in humans and mice [1] , [3] , [15] , [24] , [25] , [26] . We examined the extensor digitorum longus (EDL), which is highly enriched in fast (myosin heavy chain MyHCIIb+) myofibres; the soleus, which has >50% slow (MyHCI+) myofibres [27] , [28] and the tibialis anterior (TA), gastrocnemius and plantaris, which are composed of a range of myofibre types [27] , [28] . In addition, the diaphragm and EOMs were included because their molecular characteristics, morphology, function, innervation and aging are distinct from limb muscles [21] , [29] , [30] . We first analysed satellite cell content in sedentary 12-month-old male mice (this represents 46% of mean lifespan, based on average lifespan of 26 months for C57BL/6J mice), an age when muscle growth is complete [31] and myofibre number and CSA have not been reported to decline. Sedentary mice were chosen to represent a ‘ground’, unexercised state (without acute or intentional injuries), and only males were analysed to minimize sex-specific differences. Satellite cells were identified and quantified on sections by Pax7, a transcription factor that specifically and robustly marks satellite cells in adult and aged mice [22] , [32] . We found that most limb muscles (EDL, TA, gastrocnemius and plantaris) had similar number of satellite cells, ∼ 2,000 cells per mm 3 ( Fig. 1a–d ). The soleus and diaphragm muscles, which are enriched in slow myofibres, had 5,000 and 5,700 cells per mm 3 , respectively ( Fig. 1e,f ). EOMs had the greatest number of satellite cells, 9,800 satellite cells per mm 3 , potentially correlating with the higher density of myofibres in this muscle ( Fig. 1g ). Thus, satellite cell density varies nearly fivefold between muscles in the adult mouse. 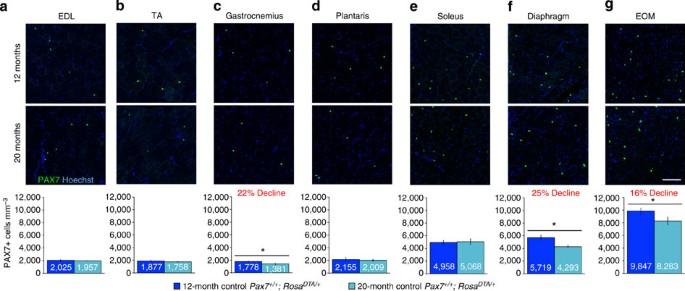Figure 1: Satellite cell number differs between muscles and with age. (a–g) Representative cross-sections showing Pax7+ satellite cells in the EDL, TA, gastrocnemius, plantaris, soleus, diaphragm and EOM muscles at 12 and 20 months in controlPax7+/+;RosaDTA/+mice. Scale bar, 100 μm. Mean number of Pax7+ satellite cells per volume (mm3) of muscle at 12 months (dark blue,n=6 EDL, TA,n=7 other muscles) and 20 months (light blue,n=3 EDL,n=5 other muscles). Data are expressed as mean±1 s.e.m. for all graphs. Two-tailed studentt-test, *P≤0.05. Figure 1: Satellite cell number differs between muscles and with age. ( a – g ) Representative cross-sections showing Pax7+ satellite cells in the EDL, TA, gastrocnemius, plantaris, soleus, diaphragm and EOM muscles at 12 and 20 months in control Pax7 +/+ ;Rosa DTA/+ mice. Scale bar, 100 μm. Mean number of Pax7+ satellite cells per volume (mm 3 ) of muscle at 12 months (dark blue, n =6 EDL, TA, n =7 other muscles) and 20 months (light blue, n =3 EDL, n =5 other muscles). Data are expressed as mean±1 s.e.m. for all graphs. Two-tailed student t -test, * P ≤0.05. Full size image To test whether satellite cell number changes over time, we quantified Pax7+ satellite cells at 20 months (77% of mean lifespan), a time at which sarcopenia of limb muscles has not been reported in mice [3] , [25] . Most limb muscles (EDL, TA, plantaris and soleus) had no change in satellite cell number at 20 months ( Fig. 1a,b,d,e ). However, in the gastrocnemius, diaphragm and EOMs, satellite cell numbers significantly declined 16–25% ( Fig. 1c,f,g ). Satellite cells contribute to myofibres in all adult muscles To test whether satellite cells contribute to myofibres during muscle homeostasis, we genetically labelled and followed the long-term fate of satellite cells in uninjured adult muscle ( Fig. 2a ). Satellite cells were labelled using Pax7 CreERT2 , an allele that we previously demonstrated specifically and efficiently induces recombination in >95% of Pax7+satellite cells after delivery of tamoxifen (TAM) [9] . We crossed these mice to the Rosa mTmG reporter, which ubiquitously expresses membrane-bound Tomato, until Cre-mediated recombination excises Tomato and results in membrane-bound green fluorescent protein (GFP) expression [33] . We generated male Pax7 CreERT2/+ ;Rosa mTmG/+ mice, labelled satellite cells at 6 months, via TAM, and harvested muscles at 12 or 20 months. In these mice, the presence of GFP+ myofibres indicates at least one satellite cell contributed to those myofibres between 6 and 12 or 6 and 20 months. In the absence of TAM, Rosa mTmG/+ mice had no GFP+ myofibres ( Supplementary Fig. 1d ) and Pax7 CreERT2/+ ;Rosa mTmG/+ mice had few GFP+ myofibres at 12 or 20 months (0–5.3% GFP/total myofibres; Supplementary Fig. 1 ), confirming that the Pax7 CreERT2 allele is tightly TAM regulated. 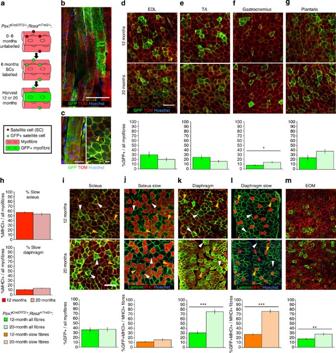Figure 2: Satellite cells contribute to myofibres in all muscles. (a) Schematic showing genetic labelling of satellite cells with GFP at 6 months and harvested at either 12 or 20 months. (b–c) GFP is broadly distributed along the length of myofibres (band left panelc) and, even in GFP myofibres, few myonuclei (orange arrow right panelc) are centrally located. (d–i,k,m) Representative cross-sections of the EDL, TA, gastrocnemius, plantaris, soleus, diaphragm and EOM of 12- or 20-month-oldPax7CreERT2/+;RosamTmG/+mice showing GFP+ myofibres to which satellite cells have contributed. It should be noted that the percentage of satellite cell contribution may be inflated in EOM due to the small size of its myofibres, which may reduce dilution of the GFP signal. Scale bar, 100 μm. (j,l) Adjacent sections in the soleus and diaphragm identifying slow MyHCI+ myofibres. White arrows indicate fast GFP+MyHCI− fibres and orange arrows indicate slow GFP+MyHCI+ fibres. Green graphs show %GFP+ myofibres at 12 months (dark green,n=4 for each muscle) or 20 months (light green,n=6 for each muscle). Orange graphs show %GFP+ MyHCI+ myofibres in the soleus (dark orange,n=4 at 12 months; light orange,n=6 at 20 months) and diaphragm (dark orange,n=3 at 12 months; light orange,n=5 at 20 months). Data are expressed as mean±1 s.e.m. for all graphs. Two-tailed studentt-test, *P≤0.05, **P<0.01 ***P<0.001. Figure 2: Satellite cells contribute to myofibres in all muscles. ( a ) Schematic showing genetic labelling of satellite cells with GFP at 6 months and harvested at either 12 or 20 months. ( b – c ) GFP is broadly distributed along the length of myofibres ( b and left panel c ) and, even in GFP myofibres, few myonuclei (orange arrow right panel c ) are centrally located. ( d – i , k , m ) Representative cross-sections of the EDL, TA, gastrocnemius, plantaris, soleus, diaphragm and EOM of 12- or 20-month-old Pax7 CreERT2/+ ;Rosa mTmG/+ mice showing GFP+ myofibres to which satellite cells have contributed. It should be noted that the percentage of satellite cell contribution may be inflated in EOM due to the small size of its myofibres, which may reduce dilution of the GFP signal. Scale bar, 100 μm. ( j , l ) Adjacent sections in the soleus and diaphragm identifying slow MyHCI+ myofibres. White arrows indicate fast GFP+MyHCI− fibres and orange arrows indicate slow GFP+MyHCI+ fibres. Green graphs show %GFP+ myofibres at 12 months (dark green, n =4 for each muscle) or 20 months (light green, n =6 for each muscle). Orange graphs show %GFP+ MyHCI+ myofibres in the soleus (dark orange, n =4 at 12 months; light orange, n =6 at 20 months) and diaphragm (dark orange, n =3 at 12 months; light orange, n =5 at 20 months). Data are expressed as mean±1 s.e.m. for all graphs. Two-tailed student t -test, * P ≤0.05, ** P <0.01 *** P <0.001. Full size image In all muscles examined at 12 or 20 months, GFP+ myofibres were present, which indicates that at least one satellite cell contributed to these myofibres ( Fig. 2 ). In longitudinal sections, GFP was often expressed along regions of the myofibre >950 μm in length ( Fig. 2b ). Given that gene products from a single myonucleus have been measured to spread 200 μm [34] and up to 1,000 μm [35] along the length of a myofibre, this suggests that potentially more than one satellite cell contributed to some GFP+ myofibres. Interestingly, while centralized myonuclei are a hallmark of satellite cell-mediated regenerated myofibres [18] , <1% of the GFP+ myofibres had centrally localized myonuclei ( Fig. 2c ). The degree of satellite cell contribution to myofibres between 6 and 12 months differed between muscles ( Fig. 2 ). In limb muscles, 8–36% of the myofibres were GFP+ ( Fig. 2d–i ), and in the diaphragm and EOM, 31 and 18% of myofibres were GFP+, respectively ( Fig. 2k,m ). Within individual muscles, the anatomical location of GFP+ myofibres varied: GFP+ myofibres were more prevalent in regions closer to the bone for the TA and gastrocnemius and in the global region of EOMs, but showed no positional bias in other muscles ( Supplementary Fig. 1 ). The diaphragm and soleus muscles contained 10 and 55% slow MyHCI+ myofibres, respectively ( Fig. 2h ). Satellite cells contributed equally to slow and fast myofibres in the diaphragm, but contributed preferentially to fast myofibres in the soleus ( Fig. 2j,l ). Thus, while satellite cells contributed to all muscles between 6 and 12 months, the degree of contribution differed between muscles, within muscles, and by fibre type. Examination of muscles at 20 months revealed that between 12 and 20 months satellite cells only continued to contribute to myofibres in a subset of muscles. In the EDL, TA, plantaris and soleus, the percentage of GFP+ myofibres did not significantly change from 12 to 20 months ( Fig. 2d,e,g,i ), indicating that satellite cells did not measurably contribute to additional myofibres after 12 months. In the gastrocnemius and EOM, the percentage of GFP+ myofibres increased ( Fig. 2f,m ), demonstrating that satellite cells contributed to an average of 1–2% of myofibres per month between 12 and 20 months (assuming continuous contribution). The diaphragm had the largest increase in GFP+ myofibres, indicating continued satellite cell contribution at a rate of 5% of myofibres per month (assuming continuous contribution; Fig. 2k ). As in the 12-month cohort, satellite cells continued to contribute equally to diaphragm slow and fast myofibres. An examination of satellite cell contribution across muscles in individual mice in the 20-month cohort revealed variability between animals: one mouse had consistently high and another mouse had consistently low levels of satellite cell contribution in multiple muscles ( P <0.003; Supplementary Fig. 2 ), despite the mice being littermates, housed together and receiving saturating levels of TAM. Together, these results demonstrate that satellite cells contribute to the myofibres of all adult muscles in the absence of injury, although the extent, distribution, rate and timing of the contribution vary between muscles and animals. By 20 months myofibres decline in size in most limb muscles myofibre CSA has been shown to decline in humans [17] , [36] , [37] and mice [3] , [15] , [25] , [38] with advanced age. Our evidence of satellite cell contribution to adult uninjured myofibres suggests that satellite cells may be important for replenishment of aging myonuclei and ultimately maintenance of myofibre CSA. We, therefore, quantified the CSA of individual myofibres in control muscles at 12 and 20 months. To quantify CSA of myofibres throughout an entire muscle, we used our newly developed analytical tool, MuscleQNT [39] . Muscles were harvested at 12 and 20 months from control male mice, sectioned and myofibres labelled with antibodies to laminin and slow MyHCI and analysed using MuscleQNT. MuscleQNT applies an adaptive thresholding method to locate myofibre boundaries and then erosion and dilation steps to isolate and quantify CSA of individual myofibres. Thus, MuscleQNT enables the unbiased, automated quantification of all myofibres in a muscle cross-section. It is best used for explicit comparison of two data sets analysed using identical input parameters, as CSA values are highly dependent on these parameters. Therefore, we analysed the sections of 12- and 20-month-old control muscles using identical input parameters (parameters for each muscle are listed in Supplementary Table 2 ). For each muscle, we generated histograms of 12- and 20-month-old myofibre CSA and determined whether the frequency of the myofibres in each bin was significantly different between 12 and 20 months via permutation tests (see Methods). We also tested for each muscle whether the overall size of myofibres was significantly different between the different aged cohorts using a hierarchical linear model with a random effect to control for intra-class correlation among measured myofibres within individual animals. Analysis at 12 months showed that myofibre size differed considerably between the muscles ( Fig. 3 ; Supplementary Fig. 3 ). The mean myofibre size in limb muscles ranged from 750 to 1,090 μm 2 ( Fig. 3a–e ; Supplementary Fig. 3a ). The mean diaphragm myofibre size was smaller (420 μm 2 ; Fig. 3f ; Supplementary Fig. 3a ), and EOM myofibres were the smallest and most tightly constrained in size (120 μm 2 ; Fig. 3g ; Supplementary Fig. 3a ). 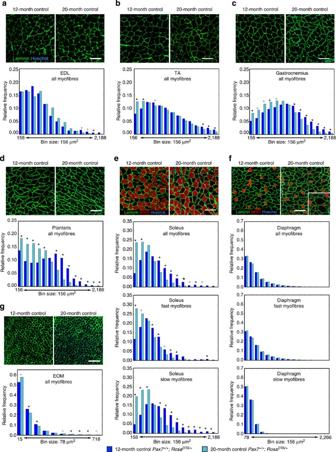Figure 3: myofibres decline in size in most limb muscles with age. (a–g) Representative cross-sections showing outlined laminin+ myofibres in the EDL, TA, gastrocnemius, plantaris, soleus, diaphragm and EOM at 12 and 20 months in controlPax7+/+;RosaDTA/+mice. Slow MyHCI+ fibres (red) are identified in the (e) soleus and (f) diaphragm. Scale bar, 100 μm for all panels. Histograms generated using MuscleQNT show relative frequency of myofibres sizes in muscles at 12 months (dark blue,n=7 for each muscle) and 20 months (light blue,n=4 for EDL,n=5 for other muscles). Additional histograms for the (e) soleus and (f) diaphragm show relative frequency of fast MyHCI− and slow MyHCI+ myofibres in muscles at 12 and 20 months. Permutation tests were conducted to determine whether counts of myofibres were significantly different in a particular bin between 12- and 20-month-old muscles (see Methods). Black asterisks indicate an empiricalP-value of <0.05 and grey asterisks a value of <0.10 (see Methods). Figure 3: myofibres decline in size in most limb muscles with age. ( a – g ) Representative cross-sections showing outlined laminin+ myofibres in the EDL, TA, gastrocnemius, plantaris, soleus, diaphragm and EOM at 12 and 20 months in control Pax7 +/+ ;Rosa DTA/+ mice. Slow MyHCI+ fibres (red) are identified in the ( e ) soleus and ( f ) diaphragm. Scale bar, 100 μm for all panels. Histograms generated using MuscleQNT show relative frequency of myofibres sizes in muscles at 12 months (dark blue, n =7 for each muscle) and 20 months (light blue, n =4 for EDL, n =5 for other muscles). Additional histograms for the ( e ) soleus and ( f ) diaphragm show relative frequency of fast MyHCI− and slow MyHCI+ myofibres in muscles at 12 and 20 months. Permutation tests were conducted to determine whether counts of myofibres were significantly different in a particular bin between 12- and 20-month-old muscles (see Methods). Black asterisks indicate an empirical P -value of <0.05 and grey asterisks a value of <0.10 (see Methods). Full size image Surprisingly, comparison of 12- and 20-month-old muscles revealed that in most limb muscles of older animals myofibres were already smaller ( Fig. 3 ; Supplementary Fig. 3 ), although in mice sarcopenia has been described as beginning at 24–26 months [3] , [15] , [24] , [26] . In the diaphragm, the distribution of myofibre sizes and average myofibre size were unaffected with age ( Fig. 3f ; Supplementary Fig. 3a ). In contrast, in the TA, gastrocnemius, plantaris and soleus, myofibres had shifted towards significantly smaller sizes ( Fig. 3b–e ; Supplementary Fig. 3a ). In the plantaris, this shift resulted in a significantly smaller total muscle CSA ( Supplementary Fig. 3b ). In the soleus, the shift to smaller myofibres occurred in both fast and slow myofibres. Finally, in the 20-month-old EOMs, the majority of myofibres shifted to smaller sizes, while a minority of myofibres hypertrophied (possibly in compensation; Fig. 3g ; Supplementary Fig. 3a ). Satellite cells are not required globally to maintain fibre CSA Our analysis unexpectedly shows that by 20 months, myofibres in most limb muscles are undergoing an age-related decline in myofibre CSA. We also find that satellite cells contribute significantly to all muscles during this time. Therefore, we hypothesized that satellite cells may be critical for the maintenance of myofibre size. If this hypothesis is correct, ablation of satellite cells should lead to smaller myofibres and potentially exacerbate the decline in CSA seen in most muscles at 20 months. To test the role of satellite cells in the maintenance of myofibre size, we genetically ablated satellite cells using Pax7 CreERT2/+ ;Rosa DTA/+ mice ( Fig. 4a ). In these mice, Cre activates the expression of diphtheria toxin A (DTA) and specifically kills Pax7+ satellite cells in response to TAM [40] , [41] . Satellite cells were ablated in male Pax7 CreERT2/+ ;Rosa DTA/+ mice via TAM at 6 months and harvested at either 12 or 20 months. Male Pax7 +/+ ;Rosa DTA/+ littermates given TAM were used as controls. In Pax7 CreERT2/+ ;Rosa DTA/+ mice given TAM, satellite cells were ablated with >97% efficiency in all muscles ( Supplementary Fig. 4 ). Again, we used MuscleQNT to analyse myofibre CSA using input parameters empirically determined for each cohort of 12- or 20-month-old control and satellite cell-ablated muscles (see parameters in Supplementary Table 2 ). 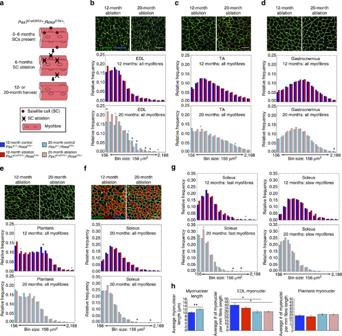Figure 4: Testing satellite cell role in maintaining size of limb myofibres. (a) Schematic showing ablation of satellite cells at 6 months and harvested at either 12 or 20 months. (b–f) Representative cross-sections showing outlined laminin+ myofibres in limb muscles EDL, TA, gastrocnemius, plantaris and soleus at 12 and 20 months inPax7CreERT2/+;RosaDTA/+mice (seeFig. 3for representative cross-sections ofPax7+/+;RosaDTA/+mice). Histograms generated using MuscleQNT show relative frequency of myofibres sizes in muscles at 12 months (dark blue, controlPax7+/+,n=7, for each muscle; red satellite cell-ablatedPax7CreERT2/+,n=8 for each muscle) and 20 months (light blue, controlPax7+/+,n=4 for EDL,n=5 for other muscles; pink, satellite cell-ablatedPax7CreERT2/+,n=6 for each muscle). Scale bar, 100 μm for all panels. (g) Additional histograms for the soleus show frequency of fast MyHCI− and slow MyHCI+ myofibres. Permutation tests (see Methods) were conducted to determine whether counts of myofibres were significantly different in a particular bin between control and satellite cell-ablated muscles. Black asterisks indicate an empiricalP-value of <0.05 and grey asterisks a value of <0.10 (see Methods). Note that the MuscleQNT parameters slightly differ between 12- and 20-month-old TA, gastrocnemius, plantaris and diaphragm muscles; to explicitly compare the CSA of 12- and 20-month-old control muscles seeFig. 3. (h) Myonuclei are significantly longer (two-tailed studentt-test, **P<0.01) and number of myonuclei are significantly reduced in 20-month versus 12-month-old EDL, but not in plantaris (two-tailed studentt-test, *P<0.05). Figure 4: Testing satellite cell role in maintaining size of limb myofibres. ( a ) Schematic showing ablation of satellite cells at 6 months and harvested at either 12 or 20 months. ( b – f ) Representative cross-sections showing outlined laminin+ myofibres in limb muscles EDL, TA, gastrocnemius, plantaris and soleus at 12 and 20 months in Pax7 CreERT2/+ ;Rosa DTA/+ mice (see Fig. 3 for representative cross-sections of Pax7 +/+ ;Rosa DTA/+ mice). Histograms generated using MuscleQNT show relative frequency of myofibres sizes in muscles at 12 months (dark blue, control Pax7 +/+ , n =7, for each muscle; red satellite cell-ablated Pax7 CreERT2 /+ , n =8 for each muscle) and 20 months (light blue, control Pax7 +/+ , n =4 for EDL, n =5 for other muscles; pink, satellite cell-ablated Pax7 CreERT2 /+ , n =6 for each muscle). Scale bar, 100 μm for all panels. ( g ) Additional histograms for the soleus show frequency of fast MyHCI− and slow MyHCI+ myofibres. Permutation tests (see Methods) were conducted to determine whether counts of myofibres were significantly different in a particular bin between control and satellite cell-ablated muscles. Black asterisks indicate an empirical P -value of <0.05 and grey asterisks a value of <0.10 (see Methods). Note that the MuscleQNT parameters slightly differ between 12- and 20-month-old TA, gastrocnemius, plantaris and diaphragm muscles; to explicitly compare the CSA of 12- and 20-month-old control muscles see Fig. 3 . ( h ) Myonuclei are significantly longer (two-tailed student t -test, ** P <0.01) and number of myonuclei are significantly reduced in 20-month versus 12-month-old EDL, but not in plantaris (two-tailed student t -test, * P <0.05). Full size image Ablation of satellite cells variably affected different muscles. In most limb muscles (TA, gastrocnemius, plantaris and soleus) at 12 or 20 months, there was no difference in average myofibre sizes or their distribution with satellite cell ablation ( Fig. 4c–g ; Supplementary Fig. 5 ). In the diaphragm, satellite cell ablation had no effect on the majority of myofibres (which are fast) at 12 or 20 months, but slow myofibres shifted to smaller sizes at 12 months ( Fig. 5a,b ; Supplementary Fig. 5 ). Interestingly, in the EOMs, satellite cell ablation had no effect at 20 months, but at 12 months resulted in smaller myofibres (seen in shift in distribution of myofibres, but not in overall average size; Fig. 5c ; Supplementary Fig. 5 ). In addition, while satellite cell ablation had no effect on the size of myofibres in the EDL at 12 months, at 20 months ablation resulted in a shift towards smaller myofibres and a significant 15% decline ( P =0.049) in average myofibre size ( Fig. 4b ; Supplementary Fig. 5 ). 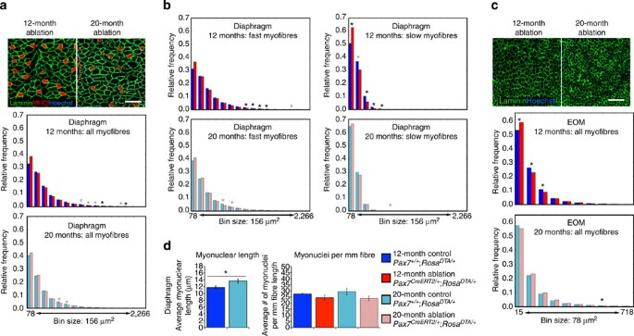Figure 5: Testing satellite cell role in maintaining EOM and diaphragm myofibres. (a,c) Representative cross-sections showing outlined laminin+ myofibres in diaphragm and EOM at 12 and 20 months inPax7CreERT2/+;RosaDTA/+mice (seeFig. 3for representative cross-sections ofPax7+/+;RosaDTA/+mice). Histograms generated using MuscleQNT show relative frequency of myofibres sizes in muscles at 12 months (dark blue, controlPax7+/+,n=7; red, satellite cell-ablatedPax7creERT2/+,n=8) and 20 months (light blue, controlPax7+/+,n=5, pink, satellite cell-ablatedPax7creERT2/+,n=6) Scale bar, 100 μm in both panels. (b) Additional histograms for the diaphragm show frequency of fast MyHCI− and slow MyHCI+ myofibres. Permutation tests (see Methods) were conducted to determine whether counts of myofibres were significantly different in a particular bin between control and satellite cell-ablated muscles. Black asterisks indicate an empiricalP-value of <0.05 and grey asterisks a value of <0.10 (see Methods). (d) Myonuclei are significantly longer at 20 months (two-tailed studentt-test, *P<0.05), but number of myonuclei do not change between 12 and 20 months in the diaphragm (two-tailed studentt-test). Figure 5: Testing satellite cell role in maintaining EOM and diaphragm myofibres. ( a , c ) Representative cross-sections showing outlined laminin+ myofibres in diaphragm and EOM at 12 and 20 months in Pax7 CreERT2/+ ;Rosa DTA/+ mice (see Fig. 3 for representative cross-sections of Pax7 +/+ ;Rosa DTA/+ mice). Histograms generated using MuscleQNT show relative frequency of myofibres sizes in muscles at 12 months (dark blue, control Pax7 +/+ , n =7; red, satellite cell-ablated Pax7 creERT2 /+ , n =8) and 20 months (light blue, control Pax7 +/+ , n =5, pink, satellite cell-ablated Pax7 creERT2 /+ , n =6) Scale bar, 100 μm in both panels. ( b ) Additional histograms for the diaphragm show frequency of fast MyHCI− and slow MyHCI+ myofibres. Permutation tests (see Methods) were conducted to determine whether counts of myofibres were significantly different in a particular bin between control and satellite cell-ablated muscles. Black asterisks indicate an empirical P -value of <0.05 and grey asterisks a value of <0.10 (see Methods). ( d ) Myonuclei are significantly longer at 20 months (two-tailed student t -test, * P <0.05), but number of myonuclei do not change between 12 and 20 months in the diaphragm (two-tailed student t -test). Full size image The observation that satellite cell ablation had an effect on the EDL, but a relatively minor effect on the diaphragm was unexpected. In the EDL, satellite cells only appreciably contributed to 30% of myofibres before 12 months. In contrast, in the diaphragm, satellite cells continuously contributed to myofibres, with 75% of myofibres having received satellite cell-derived myonuclei by 20 months. If satellite cell contribution is important for myonuclear replenishment, we reasoned that the difference in the effect of satellite cell ablation on EDL versus the diaphragm might be explained by a difference in myonuclear dynamics; satellite cell-mediated replenishment of myonuclei may only be functionally important in muscles where the number of myonuclei are declining. To test for changes in myonuclear number, we quantified the number of myonuclei in control and satellite cell-ablated diaphragms, EDL and also the plantaris (which was unaffected by satellite cell ablation, but suffered satellite cell-independent decline in myofibre CSA) at 12 and 20 months. To control for age-related changes in myonuclear size [3] , we quantified the myonuclear length from longitudinal sections of these muscles and applied a correction factor to our myonuclear counts [42] . We found that between 12 and 20 months in the diaphragm and plantaris the number of myonuclei did not decline, even in the absence of satellite cell contribution ( Figs 4h , 5d ). In contrast, in the EDL, there was a significant 25% loss of myonuclei between 12 and 20 months in control mice ( P <0.05; Fig. 4h ). The decline in myonuclei between 12 and 20 months in ablated mice demonstrates that EDL myofibres suffer myonuclear decline independent of satellite cells. However, comparison of control and satellite cell-ablated mice at either 12 or 20 months shows that the presence of satellite cells did not detectably affect myonuclear numbers in EDL myofibres. Satellite cells are the endogenous resident stem cells uniquely capable of replacing post-mitotic myonuclei and myofibres in the adult. It is well established that these stem cells are necessary and sufficient for regeneration of damaged myofibres [8] , [10] , [41] . However, satellite cells also have been hypothesized to contribute to muscle homeostasis and a decline in satellite cell-mediated replenishment of myonuclei may contribute to sarcopenia [5] , [7] . By genetically labelling and following the long-term fate of satellite cells, we demonstrate for the first time that satellite cells contribute to myofibres in all adult muscles in the absence of injury ( Fig. 6 ). The extent of this satellite cell addition varies widely between and within muscles and with age. After 12 months, satellite cells ceased to contribute to myofibres of most hind limb muscles, but not in the gastrocnemius, diaphragm and EOMs. Strikingly, only in these three muscles did the number of satellite cells decline with age. Thus, continued satellite cell contribution during homeostasis appears to deplete the pool of resident, quiescent satellite cells. 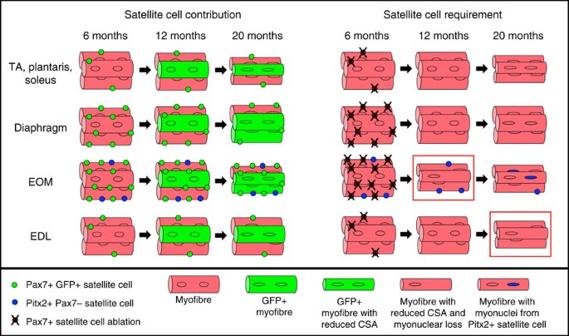Figure 6: Summary of satellite cell contribution to adult uninjured muscle. Pax7+ satellite cells, labelled at 6 months, contribute to myofibres in all muscles between 6 and 12 months. After 12 months, there is no appreciable satellite cell contribution in most limb muscles (TA, plantaris, soleus and EDL), but there is continued contribution in the diaphragm and EOM (also gastrocnemius, not shown). Pax7+ satellite cells are not required to maintain myofibre cross-sectional area of most muscles, but may help maintain myofibre CSA in EOM at 12 months and EDL at 20 months (red boxes). In EOM potentially Pax7−Pitx2+ (blue circles) satellite cells, as suggested by Hebertet al.45, compensate when Pax7+ satellites are ablated. Pax7+ satellite cells are shown as green circles in left panels and as brown circles in right panels. Figure 6: Summary of satellite cell contribution to adult uninjured muscle. Pax7+ satellite cells, labelled at 6 months, contribute to myofibres in all muscles between 6 and 12 months. After 12 months, there is no appreciable satellite cell contribution in most limb muscles (TA, plantaris, soleus and EDL), but there is continued contribution in the diaphragm and EOM (also gastrocnemius, not shown). Pax7+ satellite cells are not required to maintain myofibre cross-sectional area of most muscles, but may help maintain myofibre CSA in EOM at 12 months and EDL at 20 months (red boxes). In EOM potentially Pax7−Pitx2+ (blue circles) satellite cells, as suggested by Hebert et al . [45] , compensate when Pax7+ satellites are ablated. Pax7+ satellite cells are shown as green circles in left panels and as brown circles in right panels. Full size image The substantial contribution of satellite cells to myofibres to adult uninjured myofibres raises the question: what signals recruit satellite cells? The signal is unlikely to be myonuclear loss. Our findings that satellite cells do not contribute to EDL myofibres after 12 months despite a clear loss of myonuclei and that, conversely, satellite cells continuously contribute to diaphragm myofibres that maintain a stable number of myonuclei contradict such a hypothesis. Our data do indicate that the signals are likely to be dynamic and both local and systemic. Satellite cell contribution varies over time and between muscles, within muscles, and between fibre types, and this suggests that local signals within the muscles dynamically regulate recruitment of satellite cells. Furthermore, our observation that a few mice had higher or lower levels of satellite cell contribution across most muscles implicates the presence of systemic signals, perhaps related to the recently described G Alert signals [43] that globally modulate satellite cell recruitment to uninjured myofibres. Alternatively, this inter-animal variation may reflect differences in activity levels or other behavioural parameters. Determining the biomechanical, cellular and molecular signals regulating satellite cell recruitment will be an important area of future research. Our experiments genetically ablating satellite cells in uninjured mice explicitly test whether satellite cell contribution is critical for the maintenance of adult myofibre size ( Fig. 6 ). In most limb muscles (TA, gastrocnemius, plantaris and soleus), satellite cells were not required for the maintenance of myofibre CSA, although by 20 months these muscles suffered a satellite cell-independent decline of myofibre size. Surprisingly, despite high and continuous contribution of satellite cells to myofibres, diaphragm myofibres also did not require satellite cells for the maintenance of myofibre size (with the exception of slow myofibres, which constitute only 10% of myofibres, at 12 months). However, the stability of myonuclear numbers in the diaphragm between 12 and 20 months suggests that myonuclear replenishment may not be required during this time. A requirement for satellite cell contribution in the diaphragm and the four limb muscles may only become manifest in older (for example, 24 months) mice. EOMs are unique among the skeletal muscles in having continuous myonuclear addition throughout life [12] , [44] . Consistent with these previous reports, we found that satellite cells continuously contributed to EOM myofibres. In addition, ablation of satellite cells shifted the distribution of EOM myofibre CSA to smaller sizes at 12 months, suggesting that satellite cell contribution may be important. By 20 months, satellite cells appeared not to be required for the myofibre maintenance. However, unlike the other skeletal muscles, there is evidence that EOMs contain another population of satellite cells that are Pax7−Pitx2+ (ref. 45 ), and Pitx2 is required for the development and maintenance of EOMs [46] , [47] , [48] , [49] . Thus, this alternative Pax7− satellite cell population may compensate in the older mice lacking Pax7+ satellite cells, a hypothesis to be tested in future experiments. In mouse, the EDL is largely composed of fast MyHCIIb myofibres, and this muscle is particularly susceptible to myonuclear apoptosis, atrophy and neuromuscular dysfunction with age [15] , [50] , [51] , [52] . Consistent with these reports, we found that the EDL suffered a decline in myonuclear number between 12 and 20 months. Our lineage studies showed that satellite cells contributed to 30% of EDL myofibres before 12 months. Despite this modest contribution, ablation of satellite cells lead to a decline in myofibre CSA at 20 months. How satellite cells may play a role in maintaining EDL myofibre size is currently unclear. The most obvious hypothesis is that satellite cells replenish declining numbers of myonuclei. However, comparison of satellite cell-ablated versus control 20-month-old EDL muscles did not reveal a significant rescue of myonuclei when satellite cells were present. Satellite cells are required for regeneration and we now also show that they contribute to uninjured adult myofibres. Intriguingly, our work suggests that the mechanisms regulating satellite cells’ contribution to regenerating and uninjured myofibres may differ significantly. First, self-renewal of satellite cells is an important property of regeneration, but in muscles with continuous satellite cell contribution to uninjured myofibres the satellite cell pool is not maintained. Second, a hallmark of regenerated myofibres is the presence of centralized myonuclei. However, despite the presence of many uninjured myofibres to which satellite cells had contributed, we found few centralized myonuclei (see also ref. 22 ). Dysregulation of satellite cells may also play a role in sarcopenia. A decline in satellite cell-mediated regeneration with age has been widely recognized [23] . In addition, a decline in satellite cell contribution to uninjured myofibres may contribute to sarcopenia. Recent satellite cell ablation studies [53] found that depletion of satellite cells did not accelerate or exacerbate sarcopenia in aged mice. However, in this study, satellite cell ablation was incomplete (ranged from 64 to 87%), and in our study, we have not explicitly tested the role of satellite cells in uninjured muscle of aged (for example, 24 months) mice. Future satellite cell lineage and ablation studies of uninjured and exercised aged mice will be essential to establish whether a decline in satellite cell contribution to myofibres plays a role in sarcopenia. Mice and TAM delivery All mouse lines were previously reported: Pax7 CreERT2 (ref. 41 ); Rosa mTmG (ref. 33 ); and Rosa DTA/+ (ref. 40 ). Pax7 CreERT2 mice were backcrossed >8 generations onto C57BL/6J background. Only male mice were used, and at least five mice were used for each cohort in control and ablation studies. At 6 months of age, satellite cell-labelled ( Pax7 CreERT2/+ ;Rosa mTmG/+ , n =4 at 12 months, n =6 at 20 months), satellite cell-ablated ( Pax7 CreERT2/+ ;Rosa DTA/+ , n =8 at 12 months, n =6 at 20 months) and littermate control ( Pax7 +/+ ;Rosa DTA/+ , n =7 at 12 months, n =5 at 20 months) mice were given five 10-mg doses (50 mg total) of TAM by gavage. To ensure continuous ablation/labelling, additional 10-mg doses were given once per month until 12 months, and mice were subsequently harvested at 12 or 20 months. In addition, a small cohort of Pax7 CreERT2/+ ;Rosa mTmG/+ mice was housed separately, not given TAM and harvested at 12 or 20 months. It was noted that long-term TAM treatment led to inguinal hernias in some mice as has been reported previously [54] , though this phenotype was observed in equal ratios in control and mutant cohorts. All mice were otherwise healthy at harvest. Mice were housed in the University of Utah animal facility located at 5,000-ft elevation. No statistical method was used to predetermine sample size; all animals were included; and the experiments were not randomized. Animal experiments were performed in accordance with protocols approved by the Institutional Animal Care and Use Committee at the University of Utah. Immunofluorescence and microscopy EDL, TA, gastrocnemius, plantaris, soleus, diaphragm and EOM muscles from each animal were harvested, flash-frozen and sectioned at 8 or 12 μm (cross-sections) or 20 μm (longitudinal sections). For section immunofluorescence, slides were fixed in 4% paraformaldehyde (PFA) for 5 min, washed in 1 × PBS, and then if needed (see Supplementary Table 1 ), subjected to antigen retrieval (heated in 1.8 mM citric acid, 8.2 mM sodium citrate in H 2 0 in a 2100 PickCell Retriever). Sections that required tyramide signal amplification were quenched in 3% H 2 O 2 for 5 min. All slides were blocked in 5% serum or 0.5% TNB blocking reagent (PerkinElmer) in 1 × PBS for 60 min, and incubated in 1° antibody ( Supplementary Table 1 ) overnight at 4 °C. Slides were washed in 1 × PBS, incubated in 2° antibody 2 h at room temperature ( Supplementary Table 1 ), washed in 1 × PBS, and when needed ( Supplementary Table 1 ) incubated in Vector ABC (Vector Laboratories) for 3 h, washed in 1 × PBS and labelled with tyramide signal amplification (Fluorescein or Cy3; PerkinElmer) for 10 min. Slides were washed in PBS, post-fixed in 4% PFA, incubated with 0.4 μg ml −1 Hoechst and mounted with Fluoromount-G (SouthernBiotech). Immunofluorescent sections were imaged on a Nikon AR1 confocal or Nikon Widefield CCD Microscope. Each confocal image is a composite of maximum projections, derived from stacks of optical sections. Quantification of Pax7 and GFP contribution For the analysis of satellite cell numbers, cross-sections from the EDL, TA, gastrocnemius, plantaris, soleus, EOM and diaphragm muscles from control ( Pax7 +/+ ;Rosa DTA/+ ) and satellite cell ablation ( Pax7 CreERT2/+ ;Rosa DTA/+ ) cohorts were immunofluorescently labelled with Pax7. All Pax7+ nuclei were counted by hand (observer blinded to genotype and age), and divided by the muscle volume for each section. Volume was determined from the whole muscle CSA (using ImageJ Analyze Particles function) multiplied by the thickness of the section. To quantify satellite cell contribution to myofibres in Pax7 CreERT2/+ ;Rosa mTmG/+ mice, we immunofluorescently labelled sections for Tomato, GFP, and Hoechst and adjacent sections with MyHCI and laminin to identify slow (MyHCI+) and fast (MyHCI−) myofibres. All sections were imaged with identical exposure times and then green levels were adjusted identically in Photoshop based on the levels in control Pax7 CreERT2/+ ;Rosam mTmG.+ mice (without TAM and excluding obvious GFP+ myofibres). Only myofibres with membrane-bound GFP were counted. To quantify the percentage of GFP+ myofibres, we counted all myofibres within each muscle, and subsequently counted GFP+ fibres. For the gastrocnemius, only the lateral and intermediate muscle heads were counted, and for the diaphragm, a region containing 100 slow fibres was counted. These images were then overlaid with images from adjacent sections labelled with MyHCI and laminin to identify GFP+ slow or fast fibres (soleus and diaphragm only). All images were counted by hand, with observer blinded to age or genotype. To determine whether individual 20-month-old mice had higher or lower GFP contribution across the majority of muscles, we recorded the percentile rank of the %GFP+ myofibres in each animal in each muscle. These percentile ranks across the seven muscles for an individual mouse were used to perform t -tests (with Bonferroni correction) between animals. Quantification of myofibre CSA For analysis of myofibre CSA, we immunofluorescently labelled sections with laminin to identify myofibre borders and MyHCI to identify slow myofibres in 12- and 20-month cohorts of control Pax7 +/+ ;Rosa DTA/+ and satellite cell-ablated Pax7 CreERT2/+ ;Rosa DTA/+ mice. myofibre CSA was quantified via MuscleQNT (developed by S.F. and M.Y. and available at https://github.com/stevendflygare/muscleQNT ). MuscleQNT works by first applying an adaptive thresholding method to locate muscle fibres and then uses steps of erosion and dilation to isolate individual muscle fibres. The adaptive thresholding, erosion and dilation steps are parametric, and parameters used to score images were determined empirically (blinded to control or experimental status) for each cohort of muscles so as to best outline and isolate individual myofibres (parameters are listed in Supplementary Table 2 ). For comparison of 12- and 20-month-old control muscles ( Fig. 3 ), 12-month parameters were used (though 20-month parameters used on the same data showed identical trends, but with slightly different absolute values for fibre sizes). When using MuscleQNT, it is essential to do pairwise comparison of data sets, using exactly the same input parameters (erosion, box size, off set, minimum and maximum fibre size; Supplementary Table 2 ) as absolute CSA values are dependent on the input parameters. Once fibres are located and isolated in an image, the size of each fibre is assigned as the number of pixels it occupies. In addition, myofibres were identified as slow myofibres if more than x % ( x can be specified) of a fibre’s pixels overlap MyHCI+ pixels (colocalization function). Fibre sizes of each image are written to an output file and summary statistics generated for each image. From this data, histograms are generated comparing the distribution of myofibres between 12- and 20-month-old muscles of control and satellite cell-ablated muscles. To determine the significance of differences between 12 and 20 months or control and satellite cell-ablated muscles, permutation tests were conducted. For permutation tests, the 12- or 20-month (or control or mutant) status of the mice is randomly permuted and myofibres were randomly sampled from each of the 12/20-month-old (or control/mutant) mice. The observed differences in each histogram bin between the counts of the 12- and 20-month-old (or control and mutant) mice were recorded and compared with the differences in the corresponding histogram bins of the original 12- and 20-month-old (or control and mutant) mice. The relative proportion of times a permuted difference is as great as or greater than the observed difference in a specific histogram bin allows us to determine for a specific histogram bin the significance of the observed difference in the counts between 12- and 20-month-old (or control and mutant) mice. In addition to the analysis of the distribution of myofibre sizes, we also used a hierarchical linear regression model with a random effect to model the effect of mouse age and control/mutant status on muscle fibre size. The model leverages a random effect to control for intra-class correlation among myofibres that come from the same animal. Quantification of myonuclei The number of myonuclei per fibre for control Pax7 +/+ ;Rosa DTA/+ and satellite cell-ablated Pax7 CreERT2/+ ;Rosa DTA/+ mice for 12- and 20-month cohorts was determined using the EDL, diaphragm and plantaris cross-sections stained with laminin and Hoechst. Myonuclei were identified by their location inside the basal lamina and the number of myonuclei was counted (by an individual blinded as to section genotype and age) in the 150–250 EDL myofibres, 250–450 diaphragm myofibres and 350–525 plantaris myofibres. Myonuclear counts in cross-section can over-represent myonuclear number if myonuclei significantly change shape. To correct for this, we used a formula [42] that takes into account the observed myonuclear length in each muscle at either 12 or 20 months. We present our data as the number of myonuclei per mm of fibre length by equation (1): x = N * L /( l m + d ), where x is the number of myonuclei in a fibre segment of length L (in our case, 1 mm), N is the number of nuclei per myofibre in cross-section, l m is the average myonuclear length at 12 or 20 months and d is the thickness of the section. Myonuclear length was determined using longitudinal sections of the diaphragm and EDL (myonuclear length for EDL was used for EDL and plantaris) from Pax7 CreERT2/+ ;Rosa mTmG/+ mice harvested at 12 or 20 months. Sections were immunofluorescently labelled with GFP, laminin and Hoechst and imaged on a Nikon AR1 confocal. Optical stacks were rendered in FluoRender [55] . Myonuclei were identified by their location inside the basal lamina and measured end to end using FluoRender. For each cohort, 30 nuclei per field were analysed and average myonuclear length was determined. How to cite this article: Keefe, A.C. et al . Muscle stem cells contribute to myofibres in sedentary adult mice. Nat. Commun. 6:7087 doi: 10.1038/ncomms8087 (2015).